The splicing activator DAZAP1 integrates splicing control into MEK/Erk-regulated cell proliferation and migration Alternative splicing of pre-messenger RNA (mRNA) is a critical stage of gene regulation in response to environmental stimuli. Here we show that DAZAP1, an RNA-binding protein involved in mammalian development and spermatogenesis, promotes inclusion of weak exons through specific recognition of diverse cis -elements. The carboxy-terminal proline-rich domain of DAZAP1 interacts with and neutralizes general splicing inhibitors, and is sufficient to activate splicing when recruited to pre-mRNA. This domain is phosphorylated by the MEK/Erk (extracellular signal-regulated protein kinase) pathway and this modification is essential for the splicing regulatory activity and the nuclear/cytoplasmic translocation of DAZAP1. Using mRNA-seq, we identify endogenous splicing events regulated by DAZAP1, many of which are involved in maintaining cell growth. Knockdown or over-expression of DAZAP1 causes a cell proliferation defect. Taken together, these studies reveal a molecular mechanism that integrates splicing control into MEK/Erk-regulated cell proliferation. Alternative splicing of pre-mRNA is a key regulatory step in gene expression to increase proteome diversity in higher eukaryotes [1] , [2] , [3] , [4] . Generally, alternative splicing is regulated by multiple cis -acting splicing regulatory elements (SREs) that recruit trans -acting splicing factors to promote or inhibit the use of nearby splice sites [5] , [6] . Depending on their location and activity, the SREs are conveniently classified as exonic splicing enhancers or silencers and intronic splicing enhancers or silencersISSs). Many splicing factors function in a modular fashion with an RNA-binding module to recognize pre-mRNA and a functional module to control splicing. For example, the serine/arginine-rich (SR) proteins are known to bind ESE with RNA recognition motifs (RRMs) and promote exon inclusion with RS domains [7] , whereas the hnRNP A family can bind to enhancers splicing enhancers with RRMs and inhibit splicing with Gly-rich domains [8] , [9] . However, when recruited to intronic regions, both RS domains and Gly-rich domains can inhibit splicing [10] , [11] . Since many splicing factors have a similar domain architecture containing RNA-binding domains and low-complexity fragments, it is an intriguing idea that they may also control splicing in a modular fashion through some novel functional domains. As a key regulatory step of gene expression, alternative splicing is regulated by environmental cues through various signalling pathways that control the levels and activities of splicing factors [12] . The MEK/Erk (extracellular signal-regulated protein kinase) kinase cascade is a central component of a mitogen-activated pathway that communicates growth signals from the cell surface to the nucleus. The MEK/Erk pathway promotes cell proliferation mainly by mediating the phosphorylation of major transcription factors such as CREB and Myc to change the transcription of many targets [13] . In addition, this pathway also phosphorylates and inactivates the apoptotic regulators (for example, BAD) to control cell death [14] . It was reported that the MEK/Erk pathway affected alternative splicing of CD44 by phosphorylating and activating Sam68 (refs 15 , 16 , 17 ), and a regulatory feedback was found to link Ras activation with splicing of a different alternative exon in CD44 (ref. 18) [18] . The MEK/Erk pathway was also found to regulate the splicing of FGF receptor in response of TGF-beta stimulation [16] . In a related study, the activation of EGF was found to regulate splicing by phosphorylating SR proteins through PI3K/Akt/SRPK branch of this pathway [19] . DAZ-associated protein 1 (DAZAP1) is an hnRNP protein originally identified as binding partner of DAZ (deleted in azoospermia) [20] , [21] . It is homologous to hnRNP A1 and D family that contain two amino-terminal RRM domains followed by a low-complexity C-terminal domain (CTD) [22] ( Supplementary Fig. 1a ). DAZAP1 is highly conserved among vertebrates, with 95% amino-acid identity for the entire protein among mammals and 100% identity in the RRM region from human to frog, suggesting that it may recognize similar RNA motifs across species to control key steps in RNA metabolism ( Supplementary Fig. 1b ). DAZAP1 was shown to bind AAUAG and GU 1–3 AG in vitro but its endogenous RNA targets have not been identified on a genomic scale [23] . DAZAP1 was found in different cellular compartments depending on cell and tissue types: it is mainly localized in cytoplasm of oocytes from Xenopus or mammals [17] , [24] , but is mostly nuclear except in the elongated spermatids during spermatogenesis [20] , [25] , [26] . In cultured cells, DAZAP1 was mainly detected in nucleus but also translocated to cytoplasmic/mitochondrial compartment in response to external stimuli [27] . This protein was shown to be required in normal development and spermatogenesis in mice, as DAZAP1 deletion caused smaller body size, premature death and spermatogenesis arrest [26] . The molecular function of DAZAP1 remains unclear, although there is evidence showing that it affects mRNA localization [24] , alternative splicing [28] and translation [29] . DAZAP1 was reported to bind ESSs together with hnRNP A1/A2 in a BRCA1 exon 18 mutant and was believed to inhibit splicing [30] . In another example, DAZAP1 and hnRNP A1 were found to bind an Alu-derived fragment in an ATM intron and affect splicing in opposite ways [31] . However, the general role of DAZAP1 in regulating splicing has not been systematically studied, and its affinity for in vivo RNA substrates as well as protein interaction partners has not been examined in detail. We previously identified DAZAP1 as a binding protein for several intronic splicing enhancers or ISSs in human cells [10] , [28] . Here we thoroughly examine the direct binding of DAZAP1 to various RNA elements and to other hnRNPs, and further study the general activity of DAZAP1 in splicing regulation. We show that DAZAP1 can enhance splicing from either an intronic or exonic context, and such activity can be achieved through two mechanisms. We use mRNA-seq to identify hundreds of endogenous splicing events controlled by DAZAP1, many of which are involved in maintaining cell growth. We further study how DAZAP1 activity can be controlled through phosphorylation by the MEK/Erk pathway, and determine the function of DAZAP1 in mediating cell proliferation. Taken together, this study provides a comprehensive picture of DAZAP1-mediated splicing regulation, and reveals an integrated model that alternative splicing can be controlled through a MEK/Erk/DAZAP1 pathway to respond to outside stimuli. Intricate interaction network among RNA and hnRNPs In an unbiased screen, we identified multiple RNA motifs that function as general splicing enhancers or silencers from the intronic region [10] , [28] . Here, we use RNA affinity chromatography to identify protein factors that bind to each group of intronic splicing enhancers or silencers, and identify DAZAP1 among the binding factors for one ISE and three ISS groups (ISE group F and ISS groups F, H and I, Fig. 1a ). The RNA affinity purification also identifies other proteins in the hnRNP A1 and D family as binding partners for ISSs ( Fig. 1a ). There are two possibilities to explain the interaction between DAZAP1 with multiple RNA targets: First, DAZAP1 forms a protein–protein complex with other hnRNPs that bind to these RNA elements directly, thus DAZAP1 recognizes RNAs through a piggyback mechanism. Second, there is direct binding of DAZAP1 to different RNA elements with diverse consensus motifs. 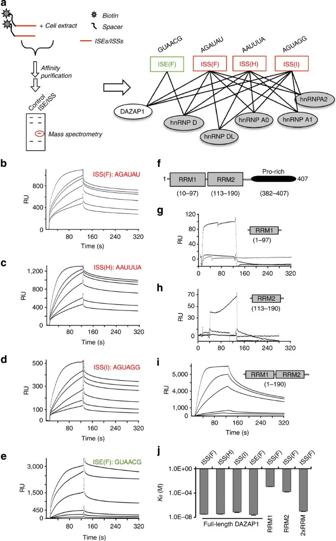Figure 1: DAZAP1 specifically interact with multiple RNA motifs. (a) Schematic diagram of RNA–protein interactions identified by affinity chromatography. The binding of different intronic SREs (ISSs or ISEs) by DAZAP1 and other hnRNPs were presented by an overlapping network. The ISE was coloured green whereas ISSs were represented in red. The representative sequence in each motif was also shown. (b–e) Full-length DAZAP1 protein interacts with four different RNA sequences as indicated above each figure. The RNA–protein interactions were measured by SPR assay using purified protein andin vitrosynthesized RNA oligos representing consensus motifs of each group. From bottom to top, the DAZAP1 concentrations were 200 nM, 300 nM, 600 nM, 1 μM, 1.5 μM and 3 μM for panelsb–d, and 60 nM, 100 nM 200 nM, 500 nM, 1 μM and 1.5 μM for panele. (f) A diagram of DAZAP1, the two RRM domains and the proline-rich CTD were shown. The recombinant proteins containing RRM domains only were constructed according to the domain annotation. (g–i) The binding of different DAZAP1 fragments (RRM1, RRM2 and both RRMs) to the cognate RNA target (ISS group F). The experimental conditions were similar to panelbexcept the protein concentrations were 1 to 5 μM for panelgandhand 50–1,000 nM for panelifrom bottom to top. (j) The bindings between different protein–RNA pairs were presented as apparent disassociation constant (Kd). All experiments were repeated three times unless indicated otherwise and error bars indicate s.d. of mean. Figure 1: DAZAP1 specifically interact with multiple RNA motifs. ( a ) Schematic diagram of RNA–protein interactions identified by affinity chromatography. The binding of different intronic SREs (ISSs or ISEs) by DAZAP1 and other hnRNPs were presented by an overlapping network. The ISE was coloured green whereas ISSs were represented in red. The representative sequence in each motif was also shown. ( b – e ) Full-length DAZAP1 protein interacts with four different RNA sequences as indicated above each figure. The RNA–protein interactions were measured by SPR assay using purified protein and in vitro synthesized RNA oligos representing consensus motifs of each group. From bottom to top, the DAZAP1 concentrations were 200 nM, 300 nM, 600 nM, 1 μM, 1.5 μM and 3 μM for panels b – d , and 60 nM, 100 nM 200 nM, 500 nM, 1 μM and 1.5 μM for panel e . ( f ) A diagram of DAZAP1, the two RRM domains and the proline-rich CTD were shown. The recombinant proteins containing RRM domains only were constructed according to the domain annotation. ( g – i ) The binding of different DAZAP1 fragments (RRM1, RRM2 and both RRMs) to the cognate RNA target (ISS group F). The experimental conditions were similar to panel b except the protein concentrations were 1 to 5 μM for panel g and h and 50–1,000 nM for panel i from bottom to top. ( j ) The bindings between different protein–RNA pairs were presented as apparent disassociation constant ( K d ). All experiments were repeated three times unless indicated otherwise and error bars indicate s.d. of mean. Full size image To distinguish these two models, we performed surface plasmon resonance (SPR) measurements to determine direct RNA–protein binding ( Fig. 1b–e ). We purified the recombinant human DAZAP1 protein to homogeneity using Ni-NTA chromatography ( Supplementary Fig. 2 ), and chemically synthesized the biotinylated RNAs representing the consensus motif of each group. We found that DAZAP1 directly binds to three ISS groups (F, H and I) and one ISE group (F) with nanomolar affinities ( Supplementary Table 1 , K d represented as mean± s.d. ), suggesting that the co-purification of DAZAP1 with intronic SREs reflected direct RNA–protein interactions. The ISS group F and H were preferably bound by DAZAP1 compared with group I, consistent with the observation that mouse DAZAP1 was shown to bind AAUAG and GU 1–3 AG sequences in vitro [23] . The three ISS groups also bind to proteins in the hnRNP A1 and D family (A0 A1 A2, D, DL) with similar affinities [10] ( Supplementary Table 1 ), consistent with our finding that the interactions between splicing factors and SREs usually form an intricate network with overlapping binding specificities [10] . DAZAP1 has two N-terminal RRMs that typically bind to single-stranded RNA in a sequence-specific manner ( Fig. 1f ); thus, we further examined if both RRMs in DAZAP1 are required for the specific RNA binding. We use the ISS group F as exemplar to measure its direct binding to the RRM1, RRM2 or both RRMs ( Fig. 1g–i ). We find that both RRMs are required for binding to the RNA target, as the individual RRM showed minimal interaction (the K d calculation was not reliable in this range). The binding affinity of 2xRRM fragment is similar to the entire protein ( Fig. 1j ). This result suggests a cooperative binding model for two RRM domains, a mechanism consistent with that of hnRNPA1 where the interdomain interaction between two RRMs is critical for RNA binding [32] , [33] , [34] . DAZAP1 interacts with proteins in the hnRNP A1 family We further examine the protein–protein interaction of DAZAP1 with other hnRNPs that copurified with DAZAP1 during the RNA affinity chromatography. Using isothermal calorimetry experiments (ITC) in the absence of RNA, we find that DAZAP1 directly interacts with purified recombinant hnRNPs (hnRNPA0, A1, A2 and D; hnRNP DL forms self-aggregates at the high concentration needed for ITC) with dissociation constant ( K d ) in micromolar range ( Fig. 2a , and Supplementary Fig. 2 ). This binding has a 1:1 stoichiometry as judged by fitting the ITC data with Langmuir binding model [35] . The bindings of DAZAP1 to other hnRNPs was mediated by the proline-rich CTD of DAZAP1, as the CTD itself had similar binding affinity to other hnRNPs as the full-length DAZAP1 ( Fig. 2b ). The N-terminal 2xRRM domain of DAZAP1 did not interact with other hnRNPs, as we fail to detect any significant binding signals using ITC assay ( Fig. 2c ). The above results suggest that the binding of DAZAP1 to hnRNPs (A0, A1, A2 or D) is mediated only by the proline-rich low-complexity CTD rather than by the RRM domains as reported previously [36] . Our finding is consistent with the reports that the low-complexity fragments in RNA-binding proteins tend to form fibres with each other [37] , [38] , [39] . The binding thermograms indicated that the protein interactions are endothermic and thus are mostly mediated through hydrophobic interactions. Consistently, it was shown that polyproline in elastin partially assumed a hydrophobic structure of polyproline II helix [40] . 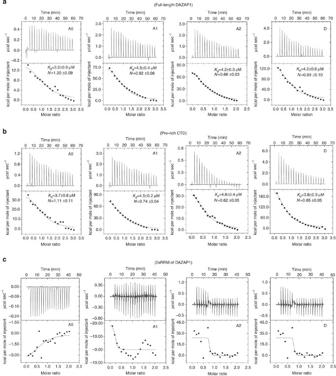Figure 2: Interaction of DAZAP1 with other hnRNPs. (a) Protein–protein interaction of full-length DAZAP1 with other hnRNPs as measured by ITC assay. All recombinant proteins were purified to homogeneity, and the DAZAP1 was titrated to purified full-length hnRNPA0, A1, A2 or hnRNP D in ITC reaction cells. Binding constants (Kd) and number of binding sites (N) were determined using by fitting the ITC data to Langmuir model. The means and ranges from two independent experiments were shown. (b) Interaction of DAZAP1 CTD with other hnRNPs as measured by ITC assay. Experimental conditions were identical to panela. (c) Lack of interaction between DAZAP1 N-terminal fragment 2xRRMs with other hnRNPs as measured by ITC assay. Experimental conditions were identical to panela. Figure 2: Interaction of DAZAP1 with other hnRNPs. ( a ) Protein–protein interaction of full-length DAZAP1 with other hnRNPs as measured by ITC assay. All recombinant proteins were purified to homogeneity, and the DAZAP1 was titrated to purified full-length hnRNPA0, A1, A2 or hnRNP D in ITC reaction cells. Binding constants ( K d ) and number of binding sites ( N ) were determined using by fitting the ITC data to Langmuir model. The means and ranges from two independent experiments were shown. ( b ) Interaction of DAZAP1 CTD with other hnRNPs as measured by ITC assay. Experimental conditions were identical to panel a . ( c ) Lack of interaction between DAZAP1 N-terminal fragment 2xRRMs with other hnRNPs as measured by ITC assay. Experimental conditions were identical to panel a . Full size image DAZAP1 promotes splicing of weak exons Since DAZAP1 interacts with multiple intronic SREs (both ISSs and ISE), we next examined if this binding could affect alternative splicing. We took advantage of a MS2 tethering system where a single MS2 hairpin site is inserted downstream of an alternative exon (exon 2 of Chinese hamster DHFR gene) [28] . The inclusion of the alternative exon is then examined with co-expression of different proteins fused with the MS2 coat protein ( Fig. 3a ). We find that when tethered into the downstream intron, DAZAP1 could promote splicing of the upstream exon as compared with the MS2 coat protein alone ( Fig. 3a ), consistent with our finding that DAZAP1 is responsible for the ISE activity in group F [28] . This activity is comparable with another splicing factor hnRNP H that is known to enhance splicing from introns ( Fig. 3a ). Interestingly, tethering of the CTD of DAZAP1 (aa 191–470) also enhances splicing with a similar activity ( Fig. 3a ), suggesting that the CTD can act as a functional domain to promote splicing from introns. 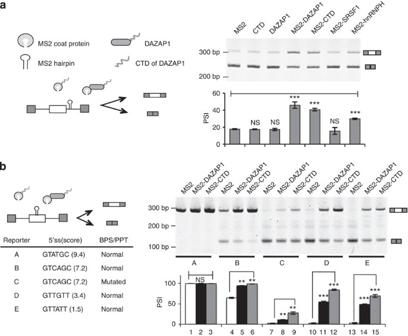Figure 3: DAZAP1 promotes splicing in exonic or intronic contexts via its CTD. (a) Schematic diagram of tethering experiments using different MS2-DAZAP1 fusion proteins and a splicing reporter (pZW2C) containing MS2 hairpin RNA in introns28. The full-length or CTD of DAZAP1 protein could promote splicing when tethered to introns. The MS2 only, CTD, and DAZAP1 alone were used as negative controls. As additional controls, two canonical splicing factors, SRSF1 and hnRNP H, were also expressed as MS2 fusion proteins. All experiments were repeated at least three times. The exon inclusion was detected by semi-quantitative RT–PCR and quantified as PSI values. The plot of mean and s.d. was shown below a representative gel.Pvalues were determined usingt-test comparing with the MS2 control. (b) Schematic diagram of tethering experiments using a series of splicing reporters with various splice site strengths and an exonic MS2 site41. The full-length or CTD of DAZAP1 fused with MS2 coat protein were shown to promote splicing for constructs B to E. All experiments were repeated three times, and a plot of mean PSI and s.d. was shown below a representative gel. In all panels, **P≤0.002; ***P≤0.001; NS, not significant (t-test). Figure 3: DAZAP1 promotes splicing in exonic or intronic contexts via its CTD. ( a ) Schematic diagram of tethering experiments using different MS2-DAZAP1 fusion proteins and a splicing reporter (pZW2C) containing MS2 hairpin RNA in introns [28] . The full-length or CTD of DAZAP1 protein could promote splicing when tethered to introns. The MS2 only, CTD, and DAZAP1 alone were used as negative controls. As additional controls, two canonical splicing factors, SRSF1 and hnRNP H, were also expressed as MS2 fusion proteins. All experiments were repeated at least three times. The exon inclusion was detected by semi-quantitative RT–PCR and quantified as PSI values. The plot of mean and s.d. was shown below a representative gel. P values were determined using t -test comparing with the MS2 control. ( b ) Schematic diagram of tethering experiments using a series of splicing reporters with various splice site strengths and an exonic MS2 site [41] . The full-length or CTD of DAZAP1 fused with MS2 coat protein were shown to promote splicing for constructs B to E. All experiments were repeated three times, and a plot of mean PSI and s.d. was shown below a representative gel. In all panels, ** P ≤0.002; *** P ≤0.001; NS, not significant ( t -test). Full size image To study how DAZAP1 was affecting splicing from an exonic context, we used a series of splicing reporters with test exons of various strengths ( Fig. 3b , reporters A to E). All reporters were inserted with an exonic MS2 site for tethering splicing factors in the test exon [41] . The co-expression of MS2-DAZAP1 enhanced the splicing of weak exons when binding to the exonic region, and this activity could be recapitulated with the CTD of DAZAP1 ( Fig. 3b ). DAZAP1 (or the CTD) had strong activity in promoting exons with a weak 5′ splice site (reporters D and E), as smaller increases were observed in the reporters with a stronger exon (reporter A and B). This 5′ splice site-dependent activity is not due to the different basal levels of exon inclusion, as the reporter C with a strong 5′ splice site but a mutated branch-point site/polypyrimidine tract had similar basal inclusion level but was weakly promoted by DAZAP1 ( Fig. 3b , lanes 7 to 9). The splice site strength-dependent activity is also found for hnRNP L and hnRNP H promoting weak exon inclusion [41] , [42] , and our findings suggest that this might be a general property for many other splicing factors. CTD of DAZAP1 binds and antagonizes hnRNPA1 The above results suggest that the proline-rich CTD of DAZAP1 is a splicing regulatory module similar to RS domains or Gly-rich domains in that it can control splicing when recruited to different pre-mRNA locations [43] . Since DAZAP1 and its CTD were found to interact with the members of hnRNP A1 family ( Fig. 2 ), we further tested if such interactions could play a role in the splicing enhancing activity of DAZAP1. The binding between DAZAP1 and hnRNP A1 was first examined in cell lysates by coimmunoprecipitation after RNase A treatment, and we find that DAZAP1 can indeed bind hnRNP A1 in cultured cells ( Fig. 4a , lane 6). In addition, this binding is mediated by interaction of the proline-rich CTD of DAZAP1 to the Gly-rich domain of hnRNP A1, as the two domains can be individually co-precipitated (lanes 7 to 9). This interaction is further confirmed with coimmunoprecipitation using endogenous DAZAP1 antibody, in which hnRNPA1, but not a control splicing factor SRSF1, is found to co-precipitate with DAZAP1 ( Supplementary Fig. 3 ). 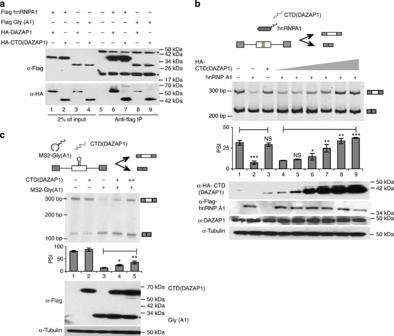Figure 4: DAZAP1 binds and antagonizes hnRNPA1 in splicing regulation. (a)In vivointeraction of DAZAP1 and hnRNP A1 as judged by coimmunoprecipitation experiments. The Flag-tagged hnRNP A1 (or Gly-rich domain of A1) and HA-tagged DAZAP1 (or its CTD) were co-expressed and pulled down using anti-Flag beads. The input and the precipitates were probed with western blots. Asterisks indicate the heavy and light chains of IgG. (b) The modular splicing reporter inserted with specific binding site of hnRNP A1 and DAZAP1 (ISS group F) in an alternative exon42was co-transfected with expression vectors of hnRNP A1 and CTD of DAZAP1 in different ratios, and the exon inclusion was detected by semi-quantitative RT–PCR and quantified. Expression vector alone was used as control (lane 1). The experiments were repeated at least three times, and the mean and s.d. were plotted below a representative gel. The protein levels were measured by western blots.Pvalues were determined with pairedt-test by comparing with lane 1 (samples 2–3) or 4 (sample 5–9). (c) The splicing reporter containing a MS2 tether site in test exon (construct B inFig. 3b) was co-transfected with the MS2 fusion protein of Gly(hnRNP A1) and the CTD of DAZAP1 in different ratios. The MS2-Gly(A1) was tethered to the splicing reporter, and the DAZAP1 CTD alone was used as additional negative control. The experiments were repeated three times, and a plot of mean and s.d. was shown below a representative gel. The protein levels were measured by western blots.Pvalues are determined witht-test by comparing lanes 4 and 5 to lane 3. In all panels, *P≤0.015; **P≤0.002; ***P≤0.0008; NS, not significant. Figure 4: DAZAP1 binds and antagonizes hnRNPA1 in splicing regulation. ( a ) In vivo interaction of DAZAP1 and hnRNP A1 as judged by coimmunoprecipitation experiments. The Flag-tagged hnRNP A1 (or Gly-rich domain of A1) and HA-tagged DAZAP1 (or its CTD) were co-expressed and pulled down using anti-Flag beads. The input and the precipitates were probed with western blots. Asterisks indicate the heavy and light chains of IgG. ( b ) The modular splicing reporter inserted with specific binding site of hnRNP A1 and DAZAP1 (ISS group F) in an alternative exon [42] was co-transfected with expression vectors of hnRNP A1 and CTD of DAZAP1 in different ratios, and the exon inclusion was detected by semi-quantitative RT–PCR and quantified. Expression vector alone was used as control (lane 1). The experiments were repeated at least three times, and the mean and s.d. were plotted below a representative gel. The protein levels were measured by western blots. P values were determined with paired t -test by comparing with lane 1 (samples 2–3) or 4 (sample 5–9). ( c ) The splicing reporter containing a MS2 tether site in test exon (construct B in Fig. 3b ) was co-transfected with the MS2 fusion protein of Gly(hnRNP A1) and the CTD of DAZAP1 in different ratios. The MS2-Gly(A1) was tethered to the splicing reporter, and the DAZAP1 CTD alone was used as additional negative control. The experiments were repeated three times, and a plot of mean and s.d. was shown below a representative gel. The protein levels were measured by western blots. P values are determined with t -test by comparing lanes 4 and 5 to lane 3. In all panels, * P ≤0.015; ** P ≤0.002; *** P ≤0.0008; NS, not significant. Full size image The results in Fig. 3 and earlier studies [28] indicate that DAZAP1 can promote splicing from both intronic and exonic locations, opposite from the activity of hnRNP A1. Therefore, we examined if the CTD domain can antagonize the splicing inhibitory activity of hnRNP A1. We use a splicing reporter with hnRNP A1-binding site (ISS group F) in an alternative exon, and co-express this with hnRNP A1 and/or the CTD of DAZAP1 ( Fig. 4b ). As expected, the hnRNP A1 alone can inhibit exon splicing, whereas the CTD of DAZAP1 alone has no effect on splicing (lanes 1 to 3, Fig. 4b ). However, the co-expression of the CTD of DAZAP1 neutralized the splicing inhibition by hnRNP A1 in a dose-dependent manner, suggesting that the binding of the CTD to hnRNP A1 can block hnRNP A1 activity. This antagonistic activity between DAZAP1 CTD and hnRNP A1 is also confirmed in endogenous genes that contain hnRNP A1/DAZAP1-binding sites near an alternative exon ( Supplementary Fig. 4 ). Because hnRNP A1 inhibits splicing through its Gly-rich domain [8] , [43] , we further tested if the direct binding of DAZAP1 CTD to this domain can revert the splicing inhibition. We tethered Gly-rich domain of hnRNPA1 to an alternative exon inserted with MS2 hairpin, and co-expressed it with the CTD of DAZAP1 ( Fig. 4c , top panel). As predicted, the MS2-Gly(hnRNP A1) inhibits splicing when recruited to the MS2 site whereas the CTD of DAZAP1 had no effect. Co-expression of the CTD (DAZAP1) with MS2-Gly(hnRNP A1) again neutralized the splicing inhibitory activity of the Gly-rich domain of hnRNP A1 in a dose-dependent manner, confirming that direct binding of these two domains plays important roles in mediating their activities ( Fig. 4c ). The Gly-rich domain of hnRNP A1 is believed to mediate the cooperative spreading of A1 along pre-mRNA [44] , [45] , and we speculate that the binding of the CTD of DAZAP1 may interfere with such spreading and thus antagonize hnRNP A1 activity. DAZAP1 regulates splicing of many genes in kinase pathways To examine how DAZAP1 affects gene expression in a global scale, we performed mRNA-seq with Illumina platform using 293 cells depleted of DAZAP1 by short hairpin RNA (shRNA) ( Fig. 5a ). By sequencing three libraries (one control and two RNA interference (RNAi) lines with different shRNAs), we obtained in total ~500 million pair-end reads of 100 nt, which were mapped to the human genome with MapSplice and further analysed with Cufflink [46] , [47] . We find that the expression levels of only four genes are significantly changed, with DAZAP1 being the most significantly decreased (with adjusted P value of 1.1E−07, Binomial test with Benjamini-Hochberg correction, Supplementary Data 1 ). In addition, two genes (MAGEA12 and ZNF804A) are significantly increased in expression and the level of one pseudogene (RP11-393N4.2) is decreased (cutoff of adjusted P value=0.05, Binomial test with Benjamini-Hochberg correction). If we relax the cutoff of the adjusted P value to 0.25, 11 genes are found to change expression levels among 17,435 genes with enough read coverage for statistical analysis (some validated in Supplementary Fig. 5 ), suggesting that DAZAP1 had little effect on gene transcription or mRNA degradation. 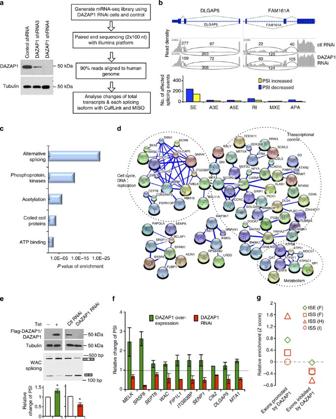Figure 5: Identification of endogenous alternative splicing events controlled by DAZAP1. (a) The 293T cells stably transfected with shRNA to knockdown DAZAP1 (left panel). The cells were subsequently used for mRNA-seq analyses as shown by schematic diagram in right panel. (b) Upper panel, two examples of alternative exons affected by DAZAP1 knockdown. The genes were chosen to show both the increase and decrease of exon inclusion, and the numbers of exon junction reads were indicated. Lower panel showed the numbers of different splicing events affected by DAZAP1 knockdown. SE, skipped exon; A3E, alternative 3′ splicing site exon; A5E, alternative 5′ splicing site exon; RI, retained intron; MXE, mutually exclusive exon; APA, alternative poly-A sites. (c) The GO analyses of DAZAP1 targets with significant splicing changes after RNAi. The Fisher ExactP-values were plotted for each enriched functional category. (d) The functional association networks of DAZAP1 targets. Genes in the categories of phosphoproteins and acetylation from panelcwere extracted and analysed with STRING database, and the interaction networks containing more than five nodes were shown. The thickness of line indicates the confidence of interactions. The gene subgroups involved in cell cycle, metabolism and transcriptional control are marked. (e) Confirmation of splicing changes for one of the DAZAP1 targets (WAC) using semi-quantitative RT–PCR in cells with over-expression or RNAi of DAZAP1. The relative changes of PSI compared with controls were calculated, and the mean and s.d. from triplicate experiments were plotted.Pvalues are calculated witht-test. *P≤0.03. (f) Validation of additional DAZAP1 targets using semi-quantitative RT–PCR in cells with over-expression or RNAi of DAZAP1. The experiments were repeated three times and the relative changes of PSI compared with controls were plotted with s.d. as error bars. For all samples,P≤0.05 in the pairedt-test by comparing PSI value of each gene with that in mock transfected controls (SeeSupplementary Fig. 6for detail). (g) Relative enrichment of RNA motifs bound by DAZAP1. Relative enrichment scores were computed for each group in the SE that were positively or negatively regulated by DAZAP1. Figure 5: Identification of endogenous alternative splicing events controlled by DAZAP1. ( a ) The 293T cells stably transfected with shRNA to knockdown DAZAP1 (left panel). The cells were subsequently used for mRNA-seq analyses as shown by schematic diagram in right panel. ( b ) Upper panel, two examples of alternative exons affected by DAZAP1 knockdown. The genes were chosen to show both the increase and decrease of exon inclusion, and the numbers of exon junction reads were indicated. Lower panel showed the numbers of different splicing events affected by DAZAP1 knockdown. SE, skipped exon; A3E, alternative 3′ splicing site exon; A5E, alternative 5′ splicing site exon; RI, retained intron; MXE, mutually exclusive exon; APA, alternative poly-A sites. ( c ) The GO analyses of DAZAP1 targets with significant splicing changes after RNAi. The Fisher Exact P -values were plotted for each enriched functional category. ( d ) The functional association networks of DAZAP1 targets. Genes in the categories of phosphoproteins and acetylation from panel c were extracted and analysed with STRING database, and the interaction networks containing more than five nodes were shown. The thickness of line indicates the confidence of interactions. The gene subgroups involved in cell cycle, metabolism and transcriptional control are marked. ( e ) Confirmation of splicing changes for one of the DAZAP1 targets (WAC) using semi-quantitative RT–PCR in cells with over-expression or RNAi of DAZAP1. The relative changes of PSI compared with controls were calculated, and the mean and s.d. from triplicate experiments were plotted. P values are calculated with t -test. * P ≤0.03. ( f ) Validation of additional DAZAP1 targets using semi-quantitative RT–PCR in cells with over-expression or RNAi of DAZAP1. The experiments were repeated three times and the relative changes of PSI compared with controls were plotted with s.d. as error bars. For all samples, P ≤0.05 in the paired t -test by comparing PSI value of each gene with that in mock transfected controls (See Supplementary Fig. 6 for detail). ( g ) Relative enrichment of RNA motifs bound by DAZAP1. Relative enrichment scores were computed for each group in the SE that were positively or negatively regulated by DAZAP1. Full size image We further examined the splicing patterns in DAZAP1 knockdown cells using the MISO package to analyse mapped reads [48] , and identify splicing events with an obvious change (≥0.1) in PSI values (percent-spliced-in) at a Bayes factor cutoff of 20. We find that a large number of alternative splicing events are significantly changed upon RNAi of DAZAP1, with the read tracks of two examples and the number of different types of events being shown ( Fig. 5b , changes of all splicing events were listed in Supplementary Data 2 ). The most abundant type of alternative splicing events affected by DAZAP1 is skipped exons. This observation that DAZAP1 mainly affects the levels of splicing isoforms rather than the total transcripts is expected, as DAZAP1 does not seem to bind DNA but rather affects RNA metabolism. We further analysed all the alternative splicing events affected by DAZAP1 using gene ontology (GO) analysis, and find that the genes affected by DAZAP1 are clustered functionally into several main groups including alternative splicing, protein phosphorylation and acetylation, gene transcription (repressors and coiled-coil domain-containing proteins), ATP binding ( Fig. 5c ). The largest group, alternative splicing, is an expected result because DAZAP1 is a splicing factor and these target genes are originally selected based on their significant change in splicing levels. Protein phosphorylation (and related ATP binding) and acetylation are the next largest functional groups, suggesting that DAZAP1 is closely involved in regulating cellular signalling pathways. We then extracted all the DAZAP1 targets in the phosphoprotein and acetylation groups, and find that many of these targets were functionally connected into well-linked interaction networks as judged by a functional network analysis using STRING (Search Tool for the Retrieval of Interacting Genes/Proteins) ( Fig. 5d ). Interestingly, the largest interaction network contained many genes in cell signalling pathways that control gene transcription, cell cycle and cell proliferation ( Fig. 5d ). This network also includes a small group of metabolic enzymes involved in ATP synthesis, suggesting that DAZAP1 may affect energy metabolism of cells. Subsequent analysis of splicing changes indicate that the splicing of ~60% of genes is positively regulated by DAZAP1 (decreased exon inclusion level or PSI value after DAZAP1 RNAi), consistent with the role of DAZAP1 to promote exon inclusion when directly binding to pre-mRNA. We further tested the results of mRNA-seq by randomly selecting several targets and assaying their splicing with reverse transcriptase polymerase chain reaction (RT–PCR) in cells with over-expression or knockdown of DAZAP1 ( Supplementary Fig. 6a,b ). As shown in the example of WAC, a gene encoding WW domain-containing adapter protein with coiled-coil to regulating H2B monoubiquitination and gene transcription [49] , DAZAP1 over-expression promotes inclusion of exon 7 to produce more full-length canonical isoforms whereas RNAi of DAZAP1 has the opposite effect ( Fig. 5e ). We further validated additional positively regulated DAZAP1 targets involved in cell proliferation and RNA processing pathways ( Fig. 5f ). For example, the SRSF6 gene encodes a splicing factor that can enhance proliferation of lung epithelial cells [50] , and MELK encodes a protein kinase that can regulate cell cycle progression by binding and phosphorylating CDC25B [51] . We obtained reciprocal splicing changes for these candidate genes in cells with over-expression and knockdown of DAZAP1 ( Fig. 5f and Supplementary Fig. 6 ), suggesting that mRNA-seq indeed can reliably identify endogenous splicing events regulated by DAZAP1. This splicing regulation activity of DAZAP1 is comparable with a well-established splicing factor SRSF1 ( Supplementary Fig. 6c ). In addition, knockdown of DAZAP1 with shRNA in HeLa cells shows similar effects on splicing of DAZAP1 targets, indicating that the splicing regulatory activity of DAZAP1 is not tissue or cell type specific ( Supplementary Fig. 6d ). We also analysed sequences around these DAZAP1-regulated exons to examine if they contain the RNA motifs recognized by DAZAP1. We extracted sequences within or at the downstream of the SE that were positively or negatively regulated by DAZAP1, and compared the relative abundance of the DAZAP1-binding motifs (three ISS groups and one ISE group) with the control exon set that were not affected by RNAi of DAZAP1. Using an enrichment score of small motifs [52] , we find, as expected, that DAZAP1-binding motifs are more enriched in exons positively regulated by DAZAP1 (that is, exon inclusion was decreased by DAZAP1 RNAi) but are slightly depleted in exons negatively regulated by DAZAP1 ( Fig. 5g ). DAZAP1 is regulated by phosphorylation through MEK/Erk DAZAP1 was shown to be phosphorylated by Erk (extracellular signal-regulated protein kinase) at two threonines (Thr269 and Thr315) in the proline-rich CTD [53] . However, the functional consequence is unclear, as this phosphorylation does not affect the ability of DAZAP1 to interact with other proteins or RNA [29] , [36] . We generated MS2 fusion proteins using a series of truncated fragments of DAZAP1 CTD, and co-expressed them with the splicing reporter containing an exonic MS2 site ( Fig. 6a , left panel). As controls, the full-length DAZAP1 and intact CTD-enhanced splicing when tethered to the exon ( Fig. 6a , constructs 1 and 2). Similarly the CTD truncations containing the two threonine phosphorylation sites can also promote splicing ( Fig. 6a constructs 3 and 4). In contrast, the truncated proteins lacking one or both of these phosphorylation sites lose their activity in enhancing splicing (lanes 5 to 7), indicating that the N-terminal fragment of the DAZAP1 CTD (including both phosphorylation sites) is critical to its activity. 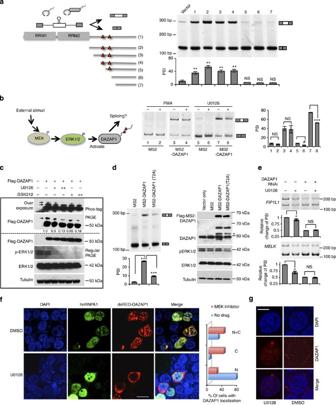Figure 6: DAZAP1 is regulated by Erk1/2 catalysed threonine phosphorylation in the CTD. (a) A series of truncated CTDs of DAZAP1 were tethered to the exon of a splicing reporter to test which regions are critical for its activity. The full-length DAZAP1 was used as positive control, and the two Erk1/2 phosphorylation sites (Thr269 and Thr315) are marked by red triangle. The experimental conditions were identical toFigure 3b. The mean PSI values and s.d. are shown below a representative gel.Pvalues were determined with pairedt-test by comparing with vector-only control. In all panels,#P≤0.05; *P≤0.01; **P≤0.002; ***P≤0.0008; NS, not significant. (b) A schematic model showing that DAZAP1 activity is mediated by MEK/Erk pathway (left panel). The tethering experiments similar to panelawere conducted in cells treated with MEK/Erk activator (PMA) or inhibitor (U0126). (c) Phosphorylation of DAZAP1 was inhibited by two specific MEK inhibitors as judged by western blot with Phos-tag labeling. The phosphorylated forms of DAZAP1 were indicated with arrows. (d) Mutation of the two DAZAP1 threonine sites phosphorylated by Erk1/2 abolished DAZAP1 activity as judged by tethering experiments. The experiments were conducted in triplicates and the mean and s.d. of PSI values are plotted below a representative gel. The western blot was shown on the right to confirm equal expression between wild-type and mutated DAZAP1. The band indicated by the asterisk is likely a degradation product of MS2-DAZAP1. (e) Inhibition of MEK/Erk by U0126 affected the splicing of endogenous DAZAP1 targets FIP1L1 and MELK. A representative gel from duplicated experiments and the relative changes of PSI were plotted with ranges as error bars. (f) Inhibition of MEK/Erk pathway affected nuclear/cytoplasmic translocation of DAZAP1. The cells were transfected with tagged DAZAP1 and hnRNP A1 and detected by corresponding antibodies. Bar, 5 μm. The percents of cells with DAZAP1 localized in nucleus (N), cytoplasm (C) or both compartments (N+C) were counted and plotted in the right panel (n=80 for each sample in two independent experiments). (g) Inhibition of MEK/Erk pathway affected nuclear/cytoplasmic translocation of endogenous DAZAP1. Scale bar, 2.5 μm. Figure 6: DAZAP1 is regulated by Erk1/2 catalysed threonine phosphorylation in the CTD. ( a ) A series of truncated CTDs of DAZAP1 were tethered to the exon of a splicing reporter to test which regions are critical for its activity. The full-length DAZAP1 was used as positive control, and the two Erk1/2 phosphorylation sites (Thr269 and Thr315) are marked by red triangle. The experimental conditions were identical to Figure 3b . The mean PSI values and s.d. are shown below a representative gel. P values were determined with paired t -test by comparing with vector-only control. In all panels, # P ≤0.05; * P ≤0.01; ** P ≤0.002; *** P ≤0.0008; NS, not significant. ( b ) A schematic model showing that DAZAP1 activity is mediated by MEK/Erk pathway (left panel). The tethering experiments similar to panel a were conducted in cells treated with MEK/Erk activator (PMA) or inhibitor (U0126). ( c ) Phosphorylation of DAZAP1 was inhibited by two specific MEK inhibitors as judged by western blot with Phos-tag labeling. The phosphorylated forms of DAZAP1 were indicated with arrows. ( d ) Mutation of the two DAZAP1 threonine sites phosphorylated by Erk1/2 abolished DAZAP1 activity as judged by tethering experiments. The experiments were conducted in triplicates and the mean and s.d. of PSI values are plotted below a representative gel. The western blot was shown on the right to confirm equal expression between wild-type and mutated DAZAP1. The band indicated by the asterisk is likely a degradation product of MS2-DAZAP1. ( e ) Inhibition of MEK/Erk by U0126 affected the splicing of endogenous DAZAP1 targets FIP1L1 and MELK. A representative gel from duplicated experiments and the relative changes of PSI were plotted with ranges as error bars. ( f ) Inhibition of MEK/Erk pathway affected nuclear/cytoplasmic translocation of DAZAP1. The cells were transfected with tagged DAZAP1 and hnRNP A1 and detected by corresponding antibodies. Bar, 5 μm. The percents of cells with DAZAP1 localized in nucleus (N), cytoplasm (C) or both compartments (N+C) were counted and plotted in the right panel ( n =80 for each sample in two independent experiments). ( g ) Inhibition of MEK/Erk pathway affected nuclear/cytoplasmic translocation of endogenous DAZAP1. Scale bar, 2.5 μm. Full size image It was previously found that the phosphorylation of DAZAP1 at Thr269 and Thr315 by Erk1/2 does not disrupt its interaction with the AU-rich RNA elements but induces its dissociation from DAZ [53] . However, this phosphorylation does not affect the translation enhancer activity of DAZAP1 (ref. 29) [29] . Given that both threonines are required for splicing activity of DAZAP1 ( Fig. 6a ), we predict that the MEK/Erk pathway can affect the splicing regulatory activity of DAZAP1 by mediating CTD phosphorylation ( Fig. 6b , right panel). To test this, we treated 293T cells with either an Erk activator (PMA, phorbol 12-myristate 13-acetate) or a well characterized MEK kinase inhibitor U0126 and determined if such treatment could affect the DAZAP1 activity in the tethering experiment ( Fig. 6b , right panel). As expected, binding of MS2-DAZAP1 to the test exon promoted splicing of that exon ( Fig. 6b , lane 1 versus 3, or lane 5 versus 7), whereas Erk activation by PMA had no obvious effect on the splicing outcome (lane 3 versus 4). However, inhibition of MEK/Erk pathway by U0126 significantly decreased the splicing activation by DAZAP1 (lane 7 versus 8), suggesting the phosphorylation of DAZAP1 by MEK/Erk is necessary for its splicing regulatory activity. Consistently, the phosphomimetic mutant of DAZAP1 (T2D; T269D/T315D) also promotes splicing, but its activity is not affected by MEK inhibition with U0126 ( Supplementary Fig. 7a ). To directly examine the phosphorylation status of DAZAP1, we used Phos-tag gels where phosphorylated proteins can be separated due to binding of Phos-tag molecules [54] . The levels of phospho-DAZAP1 species were decreased by the addition of two different MEK inhibitors, suggesting that DAZAP1 phosphorylation is mediated by MEK/Erk activation ( Fig. 6c ). Consistent with these results, we found that the mutation of the two DAZAP1 threonine sites (T2A; T269A/T315A) greatly decreased its activity in promoting the inclusion of alternative exon ( Fig. 6d ), again indicating that the threonine phosphorylation of DAZAP1 by Erk1/2 is required for its activity. In addition, the over-expression of wild-type DAZAP1 or T2D mutant, but not the T2A mutant, promoted splicing of endogenous DAZAP1 target ( Supplementary Fig. 7b ). The inhibition of MEK/Erk pathway by U0126 also decreases the splicing of the endogenous targets of DAZAP1 (FIP1L1 and MELK), and such splicing inhibition was not observed in the DAZAP1 knockdown cells ( Fig. 6e ). Taken together, these results cumulatively show that the MEK/Erk pathway controls alternative splicing through mediating the phosphorylation of a general splicing factor DAZAP1. Phosphorylation of DAZAP1 by Erk regulates its localization Like many splicing factors, DAZAP1 is known to shuttle between the nucleus and cytoplasm [20] , [27] , [55] , [56] , although it was mostly detected within the nucleus of cultured cells or spermatocytes [20] , [25] , [27] and in the cytoplasm of oocytes [17] , [24] . We further examined if the localization of DAZAP1 is affected by its phosphorylation using immunofluoresecence in cells treated with MEK inhibitors. We find that in control cells treated with DMSO, DAZAP1 localizes in the nucleus as speckled structures in the majority (~75%) of cells, whereas in some cells it can be found in both nuclear and cytoplasmic compartments ( Fig. 6f upper panels and Supplementary Fig. 8a ). Consistent with our finding, DAZAP1 also co-localizes with hnRNP A1 and A2 ( Fig. 6f and Supplementary Fig. 8c,d ), which are known nucleocytoplasmic shuttling splicing factors that interact with DAZAP1 ( Figs 2 and 4a ). Co-localization was also confirmed with antibody against endogenous DAZAP1 ( Fig. 6g , Supplementary Fig. 8c,d ). However the DAZAP1 localization is distinct from the nuclear speckles containing SC35 (SRSF2), an SR protein that promotes splicing ( Supplementary Fig. 8b ). Upon treatment with MEK inhibitor, most of the DAZAP1 proteins were localized in perinuclear/cytoplasmic regions (~80% of cells had cytoplasmic or nuclear/cytoplasmic DAZAP1 localization), while the hnRNPA1 is still found to be nuclear ( Fig. 6f ), suggesting that Erk-mediated protein translocation is specific to DAZAP1 rather than a general phenomenon for shuttling splicing factors. Serum starvation followed by the PMA treatment did not significantly alter the nuclear localization of DAZAP1 in HEK 293T cells. ( Supplementary Fig. 7c ). To further confirm this result, we mutated the two threonine residues of DAZAP1 phosphorylated by Erk1/2 and examined localization of the mutant protein. While the majority of wild-type and T2D DAZAP1 is in the nucleus, most T2A mutants are found in both the nucleus and cytoplasm ( Supplementary Fig. 9 ), which is consistent with our observations using a MEK inhibitor ( Fig. 6f ). The inefficient localization of T2A mutant in the nucleus is also consistent with our finding that this mutation decreased the DAZAP1 splicing regulation activity ( Fig. 6d ). Taken together, these results suggest that the Erk-mediated phosphorylation probably controls the splicing regulatory activity of DAZAP1 via affecting its subcellular localization. In a recent study of mouse DAZAP1, Sasaki et al . [55] found that acetylation of Lys150 in the second RRM of DAZAP1 can affect its nucleo-cytoplasmic translocation. We found that such translocation may also be regulated by phosphorylation in the CTD of DAZAP1, suggesting the subcellular localization of DAZAP1 is controlled at multiple levels through different mechanisms. DAZAP1 controls cell proliferation Because the MEK/Erk pathway plays a key role in regulating cell growth and malignant transformation, our observations suggest that DAZAP1-mediated splicing regulation might have an influence on cell growth. To test this, we generated stable cell lines with over-expressed DAZAP1 using a lung cancer cell line H157 ( Fig. 7a ) and HEK 293T cells ( Supplementary Fig. 10a ), and found that the wild-type and phosphomimetic DAZAP1 (T2D) inhibit cell growth in colony formation assays, while the T2A mutant had little effect ( Fig. 7b and Supplementary Fig. 10a ). In addition, DAZAP1 expression also decreased anchorage-independent growth of H157 cells as judged by soft agar colony assays ( Fig. 7c ). We also find that DAZAP1 can inhibit cell migration in a wound-healing assay ( Fig. 7d ), suggesting that DAZAP1-dependent splicing control may affect cell growth and migration. 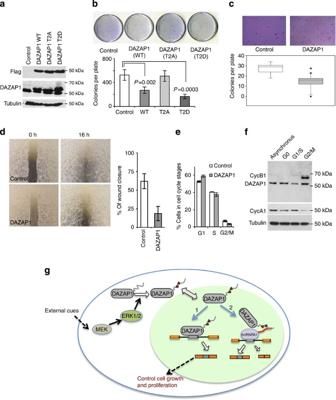Figure 7: DAZAP1 regulates cell proliferation. (a) Stable overexpression of DAZAP1 in non-small cell lung carcinoma NCI-H157 cells as detected by western blots. Control cells are stably transfected with vector only. (b) The expression of DAZAP1-inhibited cell proliferation as judged by colony formation assay with H157 cells. A representative picture from the triplicate experiments, the means and s.d. were plotted. (c) DAZAP1 inhibited the anchorage-independent cell growth of H157 as judged by soft agar assays. A representative picture from the triplicates and the quantification were shown. The box plot was drawn using 25 and 75 quartiles in Sigma Plot with whiskers indicating max and min value and dots indicating outliers.Pvalues were determined using pairedt-test, *P≤5.0 × 10−5. (d) DAZAP1 inhibited cell migration as judged by wound-healing assay. The picture of a representative plate (left panel) and the quantification of percent of gap closure were shown (right panel). Data from three independent assays were performed error bar indicate s.d. (e) The quantification of cell cycle stages (G1, S and G2/M phases) in DAZAP1 over-expressed or control cells. The cell cycle stages were analysed by flow cytometry measurement of DNA content. Data from two independent flow analysis, error bar indicate s.d. (f) Expression of endogenous DAZAP1 protein during cell cycle as detected by western blots. Tubulin and canonical cell cycle markers (cyclin A1 and B1) were also probed as controls. (g) An integrated model for DAZAP1 function and the regulation of its activity through the MEK/Erk pathway. Figure 7: DAZAP1 regulates cell proliferation. ( a ) Stable overexpression of DAZAP1 in non-small cell lung carcinoma NCI-H157 cells as detected by western blots. Control cells are stably transfected with vector only. ( b ) The expression of DAZAP1-inhibited cell proliferation as judged by colony formation assay with H157 cells. A representative picture from the triplicate experiments, the means and s.d. were plotted. ( c ) DAZAP1 inhibited the anchorage-independent cell growth of H157 as judged by soft agar assays. A representative picture from the triplicates and the quantification were shown. The box plot was drawn using 25 and 75 quartiles in Sigma Plot with whiskers indicating max and min value and dots indicating outliers. P values were determined using paired t -test, * P ≤5.0 × 10 −5 . ( d ) DAZAP1 inhibited cell migration as judged by wound-healing assay. The picture of a representative plate (left panel) and the quantification of percent of gap closure were shown (right panel). Data from three independent assays were performed error bar indicate s.d. ( e ) The quantification of cell cycle stages (G1, S and G2/M phases) in DAZAP1 over-expressed or control cells. The cell cycle stages were analysed by flow cytometry measurement of DNA content. Data from two independent flow analysis, error bar indicate s.d. ( f ) Expression of endogenous DAZAP1 protein during cell cycle as detected by western blots. Tubulin and canonical cell cycle markers (cyclin A1 and B1) were also probed as controls. ( g ) An integrated model for DAZAP1 function and the regulation of its activity through the MEK/Erk pathway. Full size image The decrease of cell growth in culture is commonly caused by increased apoptosis or disruption of cell cycle regulation, thus we tested if the DAZAP1 over-expression could affect cell cycle progression. When we measured the fractions of cells in different cell cycle stages using flow cytometry, we find that the DAZAP1 over-expression slightly increased (or did not change) the relative fraction of cells in G1 phase versus G2/M phase ( Fig. 7e ). We further used double-thymidine block to synchronize cells in different cell cycle stages, and find that DAZAP1 protein level is regulated during the cell cycle. Compared with the asynchronized culture, the DAZAP1 level is higher in G2/M phase but is decreased at the G1/S stage ( Fig. 7f ), suggesting that DAZAP1 protein expression/stability may be regulated during the cell cycle. Taken together, these data indicate that the expression level of DAZAP1 is critical to cell growth and proliferation. We initiated the mechanistic investigation of DAZAP1 by studying its interactions with RNA elements and other splicing factors. These studies further reveal its activity as a splicing activator and the underlying mechanisms of its regulation. Through a genome-wide analysis, we identify hundreds of DAZAP1-controled alternative splicing events, many of which are involved in protein phosphorylation pathways. Finally, we find that the MEK/Erk signalling pathway can control the activity and localization of DAZAP1 by mediating its phosphorylation. This study leads to an integrated model in which the MEK/Erk pathway activated by environmental cues can phosphorylate DAZAP1 to induce its translocation to the nucleus, and DAZAP1 in turn regulates cell proliferation by promoting splicing of multiple genes through two different mechanisms: by binding directly to cis -acting SREs and enhancing splicing with proline-rich CTD and by competing with and neutralizing splicing inhibitors in the hnRNP A1 family ( Fig. 7g ). DAZAP1 is found to recognize both ISSs and ISEs, causing an apparent paradox concerning how it controls splicing from introns. This paradox can be resolved by the finding that trans -acting splicing factors and cis -acting SREs usually are connected by a complex network of protein–RNA interactions rather than by one-to-one links [10] , [28] , thus the net activity of a given SRE will be a result of the integrated effect of multiple binding factors ( Fig. 1a ). Such overlapping specificities of RNA–protein interactions may provide regulatory plasticity of alternative splicing, enabling a variety of relationships including regulatory redundancy or competition [5] . In the case of DAZAP1, we show that it can promote splicing when binding to exon or introns ( Fig. 3 ). However, several DAZAP1-binding motifs (that is, three ISS groups) were also recognized by highly expressed splicing inhibitors of the hnRNP A1 family [10] , thus these motifs show splicing silencer activity despite recognition by DAZAP1. The overlap of RNA-binding specificity between splicing factors with opposite activities (for example, DAZAP1 and hnRNP A1) may also explain previous findings that the DAZAP1-binding site can function as splicing silencer in BRCA1 (ref. 30) [30] but as splicing enhancer in another case [31] . Another novel finding is that the CTD domain of DAZAP1 can promote splicing when recruited to pre-mRNA, suggesting DAZAP1 functions in a modular fashion like many transcription factors and splicing factors. The functional domain of SR proteins and hnRNP A1 were well characterized [7] , [8] , [10] , [11] , which allows the engineering of artificial splicing factors to manipulate splicing of endogenous genes [43] . Recently, the CTD of hnRNP H was identified as a new functional domain that enhances splicing when recruited to introns but inhibits splicing when tethered to exons [28] . The proline-rich CTD of DAZAP1 presented a new splicing regulatory domain that can promote splicing in exonic or intronic locations ( Fig. 3 ). This domain is directly recognized and phosphorylated by Erk1/2 kinase in two threonine sites (T269 and T315) [53] containing the TP and PxTP consensus signature of Erk substrates [57] . We demonstrate that the phosphorylation of the CTD directly affects DAZAP1 activity, as specific inhibition of MEK/Erk pathway or mutation of the DAZAP1 phosphorylation sites decreased the splicing activity of DAZAP1 ( Fig. 6b,d ). Inhibition of Erk1/2 also shows similar effects in inhibiting splicing of DAZAP1 endogenous targets ( Fig. 6e ), suggesting that the phosphorylation of the CTD of DAZAP1 is necessary for its activity. The basal level of ERK phosphorylation cannot be turned off in HEK cells even with 20 h of serum starvation ( Supplementary Fig. 11a ), thus we do not observe activation of DAZAP1 activity upon PMA treatment. However in HeLa cells where the Erk phosphorylation can be reactivated by addition of PMA, we find that the splicing of DAZAP1 targets can be further promoted by PMA treatment ( Supplementary Fig. 11b ). Taking together, these observations suggest that DAZAP1 activity is regulated by the MEK/Erk pathway, probably through phosphorylation by Erk1/2 (ref. 53) [53] . We find that the phosphorylation of DAZAP1 CTD by the MEK/Erk pathway regulates its nucleocytoplasmic translocation, which is also controlled by acetylation of lysine K150 on RRM domain [55] . Acetylation and phosphorylation often co-regulate functions of RNA-binding proteins. For example, a splicing factor SRSF2 (that is, SC35) is acetylated at the K52 of its RRM domain; such acetylation can inhibit phosphorylation of SRSF2 at the RS domain and induce its degradation [58] . The finding that DAZAP1 can be regulated by both acetylation and phosphorylation may suggest a similar bi-partite mode of post-translational modification. Our study indicates that DAZAP1 can activate splicing of alternative exons through at least two different mechanisms that may coexist in some cases. The DAZAP1 or its CTD can directly activate splicing when specifically recognizing cis -acting SREs in alternative exons or nearby introns. In addition, the DAZAP1 can also be recruited to pre-mRNA targets indirectly through binding to members of hnRNP A1 family that are well-known splicing inhibitors. The protein–protein interaction is mediated by the proline-rich CTD rather than the RRM domain of DAZAP1 ( Fig. 2 ), consistent with recent findings that low-complexity domains in many RNA-binding proteins are probably sufficient for inter- and intramolecular interaction [38] . Therefore, for pre-mRNAs with cis -elements recognized by both DAZAP1 and hnRNP A1, DAZAP1 can affect splicing through both mechanisms and the net outcome should depend on the relative protein ratio or the subtle difference of RNA affinities between these two factors. The MEK/Erk kinase cascade is a central component of the mitogenic signalling pathway. Here we show that the MEK/Erk pathway directly phosphorylates DAZAP1 and mediates its nuclear translocation and activity ( Fig. 6 ), revealing a new molecular output of the MEK/Erk pathway through regulating alternative splicing. Consistently, the endogenous targets of DAZAP1 were significantly enriched for phosphoproteins and proteins involved in acetylation or ATP binding that may play important roles in cell proliferation ( Fig. 5c ). These results identify a signalling pathway in which a splicing factor is directly controlled by MEK/Erk-mediated phosphorylation and translocation, possibly representing a new regulatory paradigm for other splicing factors. As a downstream substrate for the MEK/Erk pathway, over-expression of DAZAP1 decreased cell proliferation and migration in several assays ( Fig. 7 ). Interestingly, the knockdown of DAZAP1 also decreased cell growth without significant change in cell cycle progression ( Supplementary Fig. 10 ). These similar effects on cell growth by DAZAP1 over-expression and knockdown make the rescue experiments hard to control and interpret, suggesting the DAZAP1 levels are very critical to normal cell proliferation. It was previously reported that DAZAP1 knockout mice showed a developmental delay, small body size and slow growth rate [26] . Taken together these data suggest that the balanced level of DAZAP1 is critical for cell proliferation and has to be under tight regulation to maintain normal cell growth. Such inhibition of cell proliferation might have subtle effects on cell cycle progression ( Fig. 7e ). Apparently, DAZAP1 can delay the duration of all cell cycle stages without causing cell death. This slow growth phenotype could possibly be achieved by decreasing cell metabolism, and consistently some DAZAP1 targets are known to function in metabolic control ( Fig. 5d ). Alternatively, DAZAP1 may affect splicing of multiple genes in a balanced fashion, thus the cells can adapt to the splicing inhibition of multiple cell cycle regulators by slowing down cell growth. For example, one of the DAZAP1 targets is MELK that regulates the cell cycle by binding and phosphorylating CDC25B [51] . The DAZAP1-controlled exon skipping in MELK leads to production of an inactive isoform lacking the ATP-binding region in the kinase domain, and thus may reduce MELK activity ( Figs 5f and 6e and Supplementary Fig. 6 ). Nevertheless, the MEK/Erk/DAZAP1 pathway probably affects cell growth and migration by simultaneously shifting the splicing of multiple targets, and a thorough study of these targets will be useful in the future to provide molecular links between splicing regulation and cell proliferation. In summary, this study presents general rules of how DAZAP1 controls splicing and reveals a new function for the MEK/Erk signalling pathway. In addition to controlling transcription, the MEK/Erk pathway controls splicing and maybe other post-transcriptional RNA processing steps by mediating the translocation of DAZAP1. As an RNA-binding protein that shuttles between nucleus and cytoplasm, DAZAP1 might regulate both RNA translation (in cytoplasm) and splicing (in nucleus). Therefore, the DAZAP1 nuclear/cytoplasmic translocation controlled by the MEK/Erk pathway is critical for maintaining the homoeostasis of DAZAP1 functions. Since the MEK/Erk pathway is best known for mediating the nuclear/cytoplasmic translocation of multiple transcription factors to control cell proliferation, our findings adds yet another layer of complexity in this critical signalling pathway. Plasmid construction DAZAP1 was amplified by PCR from commercially available cDNA library (Human MTC Panel II, Clontech) using primer pair 1 and 2 ( Supplementary Table 2 ), and then subcloned into Flag-pcDNA3 vector to generate Flag-DAZAP1 construct. MS2 coat protein was amplified using primer pairs 8 and 9 using MS2-ASF as template [59] . MS2 coat protein was fused at 5′ end of either full-length DAZAP1 (aa,1–407, using primer pair 2 and 3) or DAZAP1 CTD (aa,191–407,using primer pair 2 and 7) in pcDNA3. All of the constructs were validated by sequencing. The HA-tagged version of MS2-DAZAP1/CTD was created by subcloning these amplicons into pCDNA3.1 using primer pair 2 and 11. Truncation mutants of CTD were created by PCR amplifications and followed by cloning of PCR products in pcDNAHAMS2 vector. Flag-tagged hnRNPA1 or other hnRNPs were available as a reagent from our lab [10] . All the splicing reporters were constructed from a backbone vector, pZW1 that contains a multicloning site between two GFP exons 2 (ref. 59) [59] . To construct the splicing reporter and to test function of intronic SREs, a constitutive exon—exon 6 of the human SIRT1 gene (Ensembl ID: ENSG00000096717)—was amplified together with portions of its flanking introns in two PCR reactions. The two PCR fragments were cloned into pZW1 to generate the resulting construct, pZW11, which contains a three-exon minigene with exon 1 and 3 forming an intact GFP gene and a multicloning site at 11 bp downstream of the 5′ss of the test exon 2. The candidate SRE sequences and controls were inserted into reporter pZW11 using Xho I /Apa I sites. To this end, we used a forward primer 5′-CACCTCGAG (N6) GGGCCCCAC-3′ and reverse primer 5′-GTGGGGCCC (N6) CTCGAGGTG-3′ that contained the candidate sequences (designated as ISE or ISS groups) flanked by Xho I and Apa I sites. The two primers were annealed, digested and ligated into the reporter vectors. Intronic MS2 tethering reporter was created by subcloning MS2 hairpin loop between Apa I /Xho l sites in previously described vector pZW2C [28] . The MS2 hairpin reporters (5′ss mutant and branch-point sites mutants) were created by subcloning the previously described reporter systems [41] in pcDNA3.1 between Eco R1/ Xba 1 sites (using primer pairs 17 and 18). RNA binding and SPR analysis HnRNPA0, A1, A2 D, DL and different version of DAZAP1 were cloned into pT7HTB plasmid as 6xHis-tagged protein. The recombinant proteins were expressed in Escherichia coli and purified with Ni-NTA column to homogeneity [10] . The proteins were buffer exchanged to remove excess imidazole and were stored at 4 °C for the analysis. SPR analysis was performed on Biacore 2,000 platform using biotin-labelled RNA substrates on SA-chip (GE Healthcare) [10] . The 5′-biotynalyed RNAs were synthesized by Dharmacon and immobilized at 150 fmols per flow cell on a Biacore streptavidine-coated chip (Sensor Chip SA, GE Healthcare). A control flow cell was loaded with a 21 nt CA-rich control sequence, and all the responses (RUs) were normalized to the controls. All experiments were done on Biacore 2,000 platform for at least twice in every concentration, and the data were fitted with BIAevaluation software. The protein is diluted to its final concentration by HBS-EP buffer (GE Healthcare, Cat No. BR-1001-88) prior to experiments to avoid bulk shift. Data acquisition was performed using Kinject mode at a flow rate of 50 μl min −1 in the same running buffer. The surface is regenerated using 100 μl injection of 2 M NaCl followed by 200 μl of running buffer. The data was analysed using 1:1 Langmuir model on biaevaluation software [35] . Isothermal titration experiments ITC experiment was performed on auto ITC 200 (GE Healthcare). The purified recombinant proteins were resuspended in 20 mM Na-Phosphate buffer pH 7.0 with 150 mM NaCl for ITC analysis. The full-length or truncated DAZAP1 (100–150 μM in the injection syringe) was titrated into other hnRNPs (10–15 μM of hnRNPs in the cell). Injections of 2 μl DAZAP1 protein for 20 titration points were performed and the data were fitted using Origin for ITC software. All experiments were carried out in duplicates and the average experiments were reported. Cell culture and transfection All transfection experiments were performed in HEK 293T cells unless otherwise stated. Transfection of splicing reporter constructs or protein expression vectors were carried out using Lipofectamine 2000 (Life Technologies) or lentiviral vectors as recommended by instruction manuals. The cells were co-transfected with splicing reporters and protein expression vectors, and cultured usually for 12–48 h in standard cell culture conditions as before and the samples for protein and RNA were collected. The protein was prepared using RIPA lysis buffer (Thermo Scientific), and the RNA was extracted using Trizol method (Life Technologies). To co-transfect cells with expression vectors of DAZAP1 and hnRNPA1, we used fixed amounts of Flag-tagged hnRNPA1 and increasing amounts of HA-tagged MS2 CTD of DAZAP1. The vector encoding either of the protein was transfected in ratios of (0.1:0.1; 0.1:0.2; 0.1:0.4; 0.1:0.8; 0.1:1.5; 0.1:2.0 (μg:μg)) in HEK 293T cells together with 0.2 μg splicing reporter ( Fig. 4b ). Titrations of hnRNPA1 Gly-rich domain (MS2-Gly-A1) with CTD (DAZAP1) was conducted similarly by co-transfecting fixed concentrations of Flag-MS2-Gly-A1 with increasing amounts of CTD (DAZAP1) in a ratio of 0.2:0.2 and 0.2:2.0 (μg:μg) ( Fig. 4c ). Splicing assay with semi-quantitative RT–PCR The semi-quantitative RT–PCR was performed using previously described protocols [60] . Briefly, the total RNA was purified and treated with 1U of RNAase-free DNAase (Promega) for 1 h at 37 °C, and further used as template in reverse transcription with random hexamer cDNA preparation kit (Applied Biosystem). To assay for the splicing outcome, the cDNA was amplified in 20–25 cycles using specific primer pairs in presence of Cy5–CTP (GE Healthcare). The resultant product was separated on 6% TBE-polyacrylamide (non denaturing) gel in dark and further imaged and quantified on Typhoon Trio + scanner. Immunofluorescence microscopy The dsRed-DAZAP1 construct is a gift from Dr Pauline Yen, and subsequent mutations were generated based on this construct to generate phosphorylation mutants. To detect subcellular localization of DAZAP1, cells were cultured on poly- L -lysine-coated slide and transfected with dsRed-DAZAP1 and FLAG-hnRNP A1 using lipofectamine 2000. The cells were fixed for 20 min in 4% formaldehyde 12–16 h after transfection, and permeabilized with 0.02% Triton X-100 in phosphate-buffered saline. The slides were subsequently washed and blocked with 3% BSA, and incubated with anti-Flag M2 as primary antibody (Sigma) and then with a secondary anti-mouse goat IgG (Alexa-488, Life Technologies). Microscopy was performed on Olympus confocal microscope, the pictures of at least 100 cells were captured for quantification. For endogenous protein IF 50–80% confluent cells growing on cover slips are fixed in 1% formaldehyde and essentially same steps were followed as above. Mouse hnRNPA1, hnRNPA2 and SC35 antibodies were from Santa cruz Biotech and Sigma, respectively. DAZAP1 antibody was purchased from Santacruz Biotech. The anti-mouse (Alexa-488) and anti-rabbit (Alexa-498) antibodies were from Life Technologies. All primary antibodies were used with dilution of 1:500 and fluorescent secondary antibodies were in the dilution range of 1:300 and diluted in BSA. Immunoprecipitation Standard procedures of immunoprecipitation were used. Briefly, Flag-tagged full-length hnRNPA1 or Flag-Gly(hnRNPA1) was co-expressed with HA-tagged DAZAP1 or HA-CTD-DAZAP1 in HEK 293T cells for 24 h. The cells were dislodged by trypsinization and washed with phosphate-buffered saline (DIFCO) and incubated with a lysis buffer (50 mM Tris-Cl, pH 7.4, with 150 mM NaCl, 1 mM EDTA, 1% Triton X-100 and 2 U ml −1 of RNaseA). The cell-free extract was prepared by incubating cell in the above lysis buffer for 30 min at 4 °C with occasional vortexing. Cell debris were separated by centrifugation at 15,000 r.p.m. for 15 min. M2 flag beads (20 μl, purchased from Sigma) was equilibrated on a rotary shaker using 50 mM Tris-Cl pH 7.4 with 150 mM NaCl (wash buffer). The clarified lysate was loaded on the beads and bound on rotary shaker for 2 h at 4 °C. The beads were washed with the above buffer three times and then incubated with sample buffer (125 mM Tris-Cl, pH 6.8, with 4% SDS, 20% glycerol and 0.004% bromophenol blue) at 70 °C. The samples were loaded onto SDS–PAGE gels immunoblotted and detected using anti-Flag and anti-HA antibodies. For endogenous protein IP, 50 μg anti DAZAP1 antibody (H-87: sc-67401) was immobilized onto protein A/G agarose beads (Santacruz Biotech) overnight at 4 °C on a rotary shaker. HEK 293T cells were grown in DMEM (Dulbecco's Modified Eagle Medium) media at 60–80% confluence and lysed using lysis buffer (50 mM Tris-Cl, pH 7.4, with 150 mM NaCl, 0.5% Triton X-100 and 2 U ml −1 of RNaseA and protease inhibitor). Binding and washing conditions are same as above. Elution was performed using two 70 μl 1 M glycine (pH 3.0) wash and neutralized with 1 M Tris prior to immunoblotting. Uncropped images of western blots are shown in Supplementary Fig. 12 . Phosphorylation assay Phosphorylation studies were performed on HEK 293T cells. The cells were transfected with reporter and protein expression constructs and further serum starved overnight prior to the addition of 1 μg/ml PMA (Sigma) for 40 min. The RNA was extracted using Trizol method and the splicing assay was performed as mentioned above. Addition of MEK inhibitor (U0126, Sigma) was followed 2 h post transfection and cells were collected after 16–18 h post treatment for protein and splicing analysis. The phospho-mutants were prepared using site-directed mutagenesis kit (QuikChange II kit, Merck EMD). The microscopy analysis was done on Olympus confocal microscope by counter staining the nucleus with DAPI. DAZAP1(WT) or double mutants were made as a fusion construct with pDsRed2 (Clontech, pDsRed2C1). Cells were cultured on poly- L -lysine-coated slide and transfected using Lipofectamine 2000 and fixed using 4% formaldehyde. Immunofluorescence was performed using anti-flag M2 primary antibody (Sigma, 1:1000 dilution) and subsequently detected by a secondary anti-mouse goat IgG (alexa-488, Life Technologies, 1:5000 dilution) antibody against flag-tagged hnRNPA1. Phospho-DAZAP1 was resolved on Phos-tag Gels [54] , immunoblotted and detected using anti-Flag mouse antibody (Sigma, M2 anti Flag Mouse antibody F-1804, 1:1000 dilution). Total Erk (C-16:sc-93, 1:5000 dilution), phospho Erk1/2 (E4: sc-7383, 1:3000 dilution) and DAZAP1 antibody (H-87: sc-67401, 1:5000 dilution) were from Santa Cruz Biotechnology. hnRNPA1 antibody was purchased from Cell Signaling (Cat #4296, 1:1000 dilution). HA-tagged proteins were detected using anti-mouse mAb (HRP conjugate) from Cell Signaling (cat #2999, 1:1000 dilution). Uncropped images of western blots are shown in Supplementary Fig. 12 . High throughput sequencing and analysis Cell lines stably transfected with shRNA 3 (5′- CCGG CAGGGAATACTTCAAGAAGTT CTCGAGAACTTCTTGAAGTATTCCCTGTTTTTG-3′ ) or shRNA4 (5′- CCGG CCCAGGAGCGATAACAGTAAACTCGAGTTTACTGTTATCGCTCCTGGGTTTTTTG -3′) vector (cloned into pLKO.1 TRC cloning plasmid) against DAZAP1 were created. Total RNA from shRNA knockdown lines or a mock transfected lines were purified using Trizol method and subsequently cleaned using RNAeasy Kit (Qiagen) the bound RNA digested with RNAse free DNAse in column as per manufacturer’s instruction. Total RNA not exceeding 3 μg was further used to purify poly-A RNA using Illumina TruSeq Total RNA Sample Prep kits with Ribo-Zero Human for removal of cytoplasmic rRNA. The mRNA purified was further analysed using Bioanalyzer (Agilent Technologies) prior to generation of cDNA with bar coded ends. The TruSeq SR Cluster Kit v3-cBot-HS was next used to cluster generation reagents for the cBot cluster amplification system in a pre-mixed, 96-well plate format that requires minimal reagent preparation. The cluster generation and sequencing were carried out by standard procedures in HiSeq 2000 Illumina platform, and we used paired-end sequencing protocol to generate 100 nt read at each end. The paired-end sequences were aligned against human genome (hg19) using MapSplice 2.0.1.6 (default parameters) to discover splicing junctions [46] . The alignments were then further analysed by Cufflinks 2.0.2 to calculate the abundance (FPKM) of genes and transcripts. The change of splicing isoforms were analysed using MISO package with the annotation of all known alternative splicing events [48] , and we filtered the results based on the Bayes Factor and PSI (percent-spliced-in) values. The GO analysis was performed using DAVID GO analysis software to search for enriched pathways. The genes in categories of phosphoproteins and acetylation from GO analysis were extracted and analysed with STRING database, and the networks containing more than five nodes were analyses for their function annotations. A number of the targets enriched in our screen were tested for splicing changes by semi-quantitative RT–PCR analysis as described earlier. To analyse the enrichment of DAZAP1 target motifs in endogenous targets, we extracted the SE that were significantly affected by RNAi of DAZAP1. The alternative exons were classified according to the changes of PSI value into three categories: exons positively regulated by DAZAP1 (PSI value decreased by at least 0.1 upon RNAi of DAZAP1), exons negatively regulated by DAZAP1 (PSI value increased by at least 0.1 upon RNAi of DAZAP1) and exons unaffected by DAZAP1 (PSI value changed by less than 0.1). The exonic sequences and 400 nt intronic sequence at the downstream of exons were extracted for each class, and we used a standard score (RESCUE score) [52] to measure the enrichment of each SRE motifs. Generation of stable cell lines Cell culture was performed on standard DMEM media supplemented with 10% fetal bovine serum (FBS) (Life Technologies) with exception of NCI-H157 cell that were maintained on RPMI (Sigma) media supplemented with 10% FBS. To generate stable lines over-expressing Flag-DAZAP1, the cDNA was cloned in pCDH expression plasmid (System Biosciences) and was further transfected to HEK 293T cells to generate virus. The supernatant media from the same culture was further clarified by centrifugation to remove any cellular contaminant and used for infecting cell lines of interest. The infected cells were selected for stable integrants in puromycin-containing media for at least three generations, prior to screening by western blot for the production of Flag-tagged DAZAP1 product. The knockdown lines of DAZAP1 were made by cloning stable hairpin structure targeting DAZAP1 coding region (5′-CAGGGAATACTTCAAGAAGTT-3′) in pLKO.1 TRC cloning plasmid (Addgene). The shRNA-containing virus was made in HEK 293T cells, and transduction was performed using standard manufacturer’s instruction. The shRNA lines were selected for 2 weeks on puromycin-containing media and the reduction of DAZAP1 was confirmed by western blot. Tetracycline-inducible DAZAP1 lines in HEK 293T cells were generated and maintained as described previously [28] . Cell proliferation assay and cancer cell growth Colony formation assay was performed by plating equal amount of cell on 100 cm tissue culture dish in DMEM media containing 10% FBS, the culture was followed for 2 weeks and fixed using 2% formaldehyde and stained with crystal violet solution at room temperature. The dried plates were used for estimation of colony diameter and number. Scratch healing assay was performed using standard protocol [61] and quantified using IMAGEJ software. Soft agar invasion assay was performed by plating 2 × 10 4 cells on 6-well dishes 0.35% BD Difco Noble agar (BD Diagnostic Systems) over a bottom layer of 0.5% BD DIFCO Noble agar containing RPMI, respectively. Cultures were maintained for a minimum of 4 weeks by weekly addition of fresh media to the top layer, cells were then stained with Crystal violet and imaged. For flow cytometry analysis, cells growing in early stationary stage was collected and fixed using cold 70% ethanol and further stained with PI with RNAse (BD Pharmingen). Cell cycle analysis was performed using CyAn ADP Analyzer Flow Cytometer (Beckman Coulter) and analysed using Mod Fit analysis software (Variety software house). Statistical analysis Statistical significance was tested by t -test or paired t -test using the Sigma Plot Software (Systat). Accession codes: RNA sequencing data have been deposited in Gene Expression Omnibus database (accession number GSE52745 ). How to cite this article: Choudhury, R. et al. The splicing activator DAZAP1 integrates splicing control into MEK/Erk-regulated cell proliferation and migration. Nat. Commun. 5:3078 doi: 10.1038/ncomms4078 (2014).